NAD+protects against EAE by regulating CD4+T-cell differentiation CD4 + T cells are involved in the development of autoimmunity, including multiple sclerosis (MS). Here we show that nicotinamide adenine dinucleotide (NAD + ) blocks experimental autoimmune encephalomyelitis (EAE), a mouse model of MS, by inducing immune homeostasis through CD4 + IFNγ + IL-10 + T cells and reverses disease progression by restoring tissue integrity via remyelination and neuroregeneration. We show that NAD + regulates CD4 + T-cell differentiation through tryptophan hydroxylase-1 ( Tph1 ), independently of well-established transcription factors. In the presence of NAD + , the frequency of T-bet −/− CD4 + IFNγ + T cells was twofold higher than wild-type CD4 + T cells cultured in conventional T helper 1 polarizing conditions. Our findings unravel a new pathway orchestrating CD4 + T-cell differentiation and demonstrate that NAD + may serve as a powerful therapeutic agent for the treatment of autoimmune and other diseases. CD4 + T helper (Th) cells play a central role in regulating the adaptive immune response associated with pathogen invasion. To date, several CD4 + Th cell subsets have been described. Th1 and Th2 subsets were the first described [1] , [2] , [3] , [4] , whereas Th17 and induced regulatory T cells were characterized more recently [5] , [6] , [7] . Each distinct CD4 + T-cell subset has a specific function and can mainly be distinguished by its cytokine profile, the expression pattern of cell surface molecules, and the activation of specific transcription factors [8] . However, the function of CD4 + T cells can be impaired resulting in numerous diseases, including allergic responses, tumour immunity and autoimmunity [9] , [10] . In multiple sclerosis (MS), Th1 and Th17 subsets have been shown to play a central role [11] . MS is an inflammatory-mediated demyelinating disease that has been associated with production of interferon (IFN)-γ and interleukin (IL)-17, two cytokines that are produced by Th1 and Th17 cells, respectively [12] . More recently, the role of Th1 and Th17 CD4 + cells in the pathogenesis of experimental autoimmune encephalomyelitis (EAE), the most commonly used experimental model for human MS, has been challenged, and it has been demonstrated that the transcription factor T-bet (also known as Tbx21 ) is critical for controlling Th1/Th17-mediated autoimmunity [12] . In contrast, regulatory T cells (Tregs) play a cardinal role in protecting against autoimmune diseases, inflammation and tissue damage [13] through secretion of IL-10 (ref. 14 ) and other mechanisms. Although differentiation of naïve CD4 + T cells has been considered to be an irreversible process, accumulating evidence suggests that T cells are much more flexible than initially believed with the ability to interchange between helper phenotypes [15] . For instance, Th17 cells are able to co-produce IFN-γ, initially considered exclusively a Th1 cytokine [16] , [17] . It has been shown that Th17 cells can also co-express Foxp3 or T-bet [18] , [19] , which are the master regulators of Tregs and Th1 cells, respectively. Moreover, Th1 IFN-γ-producing cells have been shown to have the capacity to produce the immunosuppressive cytokine IL-10, initially considered a Th2 cytokine [20] . Studies have shown that Th1 IFN-γ-producing cells that co-produce IL-10 have immunosuppressive properties and can protect from tissue damage [21] , [22] . In addition, it was recently shown that Th17 cells that were generated with transforming growth factor (TGF)-β and IL-6 were not pathogenic and did not induce EAE without exposure to IL-23 (ref. 23 ). Thus, these reports suggest the existence of broad plasticity of Th1 and Th17 cells. In EAE, it was reported that nicotinamide (Nam), a precursor of nicotinamide adenine dinucleotide (NAD + ) biosynthesis, plays an important role in the disease. This study reported that Nam reduced CD4 + T cell infiltration and demyelination [24] , but failed to identify the protective mechanisms of action. In contrast, a different study found that inhibition of NAD + synthesis by FK866, an inhibitor of nicotinamide phosphoribosyltransferase (Nampt), protected against EAE [25] . In this latter study, it was reported that FK866 treatment was associated with a massive depletion of NAD + in activated CD3 + T lymphocytes and impaired their proliferation and cytokine production [25] . Furthermore, numerous studies have underscored the role of NAD + , a co-factor found in all living cells and in nutrients, in T-cell regulation. In vivo , NAD + has been shown to induce apoptosis in naïve CD4 + CD62L high T cells and Foxp3 + regulatory T cells [26] , [27] . Conversely, activated CD44 high CD69 high T cells were more resistant to NAD + -induced cell death [26] . Moreover, it was reported that NAD + regulates cytokine production of peripheral blood lymphocytes and monocytes [25] , [28] . These studies provided a strong rationale to investigate the role of NAD + in CD4 + T cells and its impact on EAE. Here we show that administration of NAD + protects against EAE and reverses disease progression by regulating CD4 + T-cell differentiation and apoptosis through a novel signalling pathway and by promoting myelin and axonal regeneration. NAD + restores tissue integrity and induces homeostasis Increasing evidence indicates that NAD + may play an active role in protecting against EAE [24] , [29] . Consequently, we used the widely utilized EAE mouse model that recapitulates human MS, to study the impact of NAD + on EAE. Our results showed that onset of clinical signs of EAE in mice injected with myelin olygodendrocyte glycoprotein (MOG) peptide occurred after 11 days, and severe EAE was exhibited after 18 days with bilateral hindlimb paralysis ( Fig. 1a and Supplementary Movie 1a and 1b ). In contrast, mice treated daily with NAD + were protected against EAE and exhibited no signs of paralysis ( Fig. 1a and Supplementary Movie 1c ). Moreover, NAD + -treated mice did not develop EAE even after 25 days ( Fig. 1a and Supplementary Movie 1f ), whereas non-treated mice exhibited severe symptoms ( Fig. 1a and Supplementary Movie 1d ). Furthermore, to assess the clinical efficacy of NAD + and its therapeutic potential, a group of mice that had developed severe clinical symptoms of EAE (that is, bilateral hindlimb paralysis) was subjected to daily NAD + treatment starting 15 days after MOG immunization. As shown in Fig. 1a and Supplementary Movie 1e , daily treatment with NAD + starting 15 days after MOG immunization reversed the progression of the disease when compared with the group of mice that had been treated with a placebo solution ( Fig. 1a and Supplementary Movie 1d and e ). Treatment with NAD + starting 15 days after MOG immunization rapidly resolved (within 10 days of treatment) the bilateral hindlimb paralysis, whereas a majority of the non-treated mice continued to exhibit bilateral hindlimb paralysis or weakness ( Fig. 1a and Supplementary Movie 1d and 1e ). Taken together, these results indicate that NAD + treatment is not only able to block EAE progression, but can also rapidly reverse it. Thus, we next investigated how NAD + treatment was able to arrest and reverse EAE progression and assessed whether NAD + was able to reverse the clinical symptoms of EAE by protecting axons from degeneration and whether NAD + had the capacity to promote myelin regeneration. Luxol fast blue (LFB) staining showed dramatic myelin loss, and haematoxylin and eosin (H&E) staining revealed extensive inflammatory infiltrates of mononuclear cells in the spinal cords of mice treated with a placebo solution ( Fig. 1b,e ). In contrast, the spinal cords of mice treated daily with NAD + remained free of myelin loss and inflammatory infiltrates ( Fig. 1c,f ) in LFB and H&E staining. More importantly, the spinal cords of mice treated with NAD + starting 15 days after MOG immunization (that is, treated after hindlimb paralysis) did not show myelin loss and inflammatory infiltrate ( Fig. 1d,g ) in LFB and H&E staining. In addition, demyelination and axon loss were assessed with antibodies to myelin basic protein (MBP/SMI-9) and neurofilament (NF) 200, respectively, in all three groups ( Fig. 1b–g ). Consistent with H&E and LFB findings, a significant reduction in both MBP staining depicting demyelination and axon loss evidenced by reduced NF 200 staining was very prominent in the group of mice treated with a placebo solution ( Fig. 1b,e ) when compared with the daily NAD + -treated group ( Fig. 1c,f ) and with mice treated with NAD + after developing hindlimb paralysis (15 days after MOG immunization; Fig. 1d,g ). Furthermore, areas and degree of demyelination and axon loss were quantified in mice treated with placebo solution and the group of mice treated with NAD + daily or 15 days after MOG immunization ( Fig. 1h,i ). The results indicated a higher optical density of LFB and NF immunofluorescence in the two groups of NAD + -treated mice when compared with the control group ( Fig. 1h,i ). Of note, optical density of LFB immunostaining was more pronounced in the group of mice treated with NAD + daily when compared with the late-treated group; this was less pronounced in the NF immunofluorescence ( Fig. 1h,i ). A recent study has shown that NAD + precursor Nam) plays an important role in governing stem cell pluripotency [30] . In the adult spinal cord, neural stem cells have been reported to reside close to the central canal—in the ependymal layer [31] , [32] , subependymally [33] or in the white matter parenchyma [34] . In mice treated daily with NAD + , the ependymal cell population showed significant Ki67 immunoreactivity indicating ependymal proliferation when compared with mice treated with placebo solution ( Fig. 1j ). Ependymal cells were also strongly immunoreactive for neural stem cell marker Musashi upon NAD + treatment when compared with the respective control ( Fig. 1k ). Increased Ki67 and Musashi labelling were also observed subependymally and in the outer white matter in NAD + -treated spinal cords ( Supplementary Fig. 1 ). Collectively, these results indicate that NAD + blocks EAE progression by protecting against myelin and axonal damage, and more importantly, that NAD + reverses EAE progression by promoting myelin and axonal regeneration. 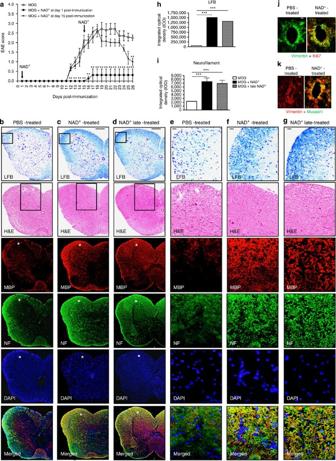Figure 1: NAD+prevents demyelination and axon loss. (a) Behavioural scores of EAE in C57BL/6 mice treated at the day of MOG immunization daily with intraperitoneal injection of 60 mg of NAD+or a placebo solution (PBS). An additional group of mice was treated with intraperitoneal injection of 60 mg of NAD+15 days after MOG immunization (n=8–11 per group). (b–i) Myelin and neurofilament (NF) assessment in spinal cord of: (b) mice that were treated daily with a placebo solution (PBS), (c) mice that were treated daily with NAD+and (d) mice that were treated with NAD+15 days after MOG immunization (when mice developed hindlimb paralysis). (b–d) Paraffin sections were stained with luxol fast blue (LFB) to assess demyelination, H&E for lymphocyte infiltration, myelin basic protein (MBP) to assess demyelination, NF 200 for axon loss and DAPI to label nuclei. Merged images of MBP, NF and DAPI are also shown. The boxed regions ina–cfor LFB and H&E staining have been magnified ind–f, respectively. The white stars ina–cfor MBP, NF, DAPI and merged images depict regions that are shown in higher magnification ind–f. Scale bars:a, 100 μm (applies tob–d),d, 50 μm (applies toe–g). (h,i) Quantification of myelination and NF-positive areas showing a significant protection and recovery of (h) myelin and (i) NFs following daily NAD+treatment and administration 15 days after MOG immunization. (j,k) Vimentin/Ki67 (j) and Vimentin/Musashi (k) co-labelling revealed increased ependymal cell proliferation in NAD+-treated spinal cord when compared with PBS-treated spinal cord. Scale bars: (b), 100 μm (applies toc,d); (e), 50 μm (applies tof,g); (j), 20 μm (applies tok);n=8–11; data derived from three independent experiments. Data represent mean±s.d. *P<0.05; **P<0.01; ***P<0.001, NS, not significant. Student’st-test and Mann–WhitneyU-test were used accordingly to compare between groups. Figure 1: NAD + prevents demyelination and axon loss. ( a ) Behavioural scores of EAE in C57BL/6 mice treated at the day of MOG immunization daily with intraperitoneal injection of 60 mg of NAD + or a placebo solution (PBS). An additional group of mice was treated with intraperitoneal injection of 60 mg of NAD + 15 days after MOG immunization ( n =8–11 per group). ( b – i ) Myelin and neurofilament (NF) assessment in spinal cord of: ( b ) mice that were treated daily with a placebo solution (PBS), ( c ) mice that were treated daily with NAD + and ( d ) mice that were treated with NAD + 15 days after MOG immunization (when mice developed hindlimb paralysis). ( b – d ) Paraffin sections were stained with luxol fast blue (LFB) to assess demyelination, H&E for lymphocyte infiltration, myelin basic protein (MBP) to assess demyelination, NF 200 for axon loss and DAPI to label nuclei. Merged images of MBP, NF and DAPI are also shown. The boxed regions in a – c for LFB and H&E staining have been magnified in d – f , respectively. The white stars in a – c for MBP, NF, DAPI and merged images depict regions that are shown in higher magnification in d – f . Scale bars: a , 100 μm (applies to b – d ), d , 50 μm (applies to e – g ). ( h , i ) Quantification of myelination and NF-positive areas showing a significant protection and recovery of ( h ) myelin and ( i ) NFs following daily NAD + treatment and administration 15 days after MOG immunization. ( j , k ) Vimentin/Ki67 ( j ) and Vimentin/Musashi ( k ) co-labelling revealed increased ependymal cell proliferation in NAD + -treated spinal cord when compared with PBS-treated spinal cord. Scale bars: ( b ), 100 μm (applies to c , d ); ( e ), 50 μm (applies to f , g ); ( j ), 20 μm (applies to k ); n =8–11; data derived from three independent experiments. Data represent mean±s.d. * P <0.05; ** P <0.01; *** P <0.001, NS, not significant. Student’s t -test and Mann–Whitney U -test were used accordingly to compare between groups. Full size image EAE is a well-established mouse model that mimics many important features of MS in humans including the immune response. It is well established that Th1 and Th17 CD4 + cells play a critical role in the pathogenesis of EAE, and the transcription factor T-bet has been shown to play a critical role in controlling Th1/Th17-mediated autoimmunity [12] . In contrast, Tregs and IL-10 have been shown to play a major role in protection against and recovery from EAE [35] . Our results demonstrate that NAD + acts on the central nervous system (CNS) by promoting myelin and axonal regeneration. However, its role on the immune response in EAE remains unknown. Thus, we next investigated whether NAD + treatment protected against EAE by modifying the systemic immune response. Consistent with a previous report [27] , we found that NAD + treatment reduced the number of CD4 + CD25 + Foxp3 + cells ( Fig. 2a ). Furthermore, although mice treated with NAD + were resistant to EAE, we found that NAD + promoted a robust Th17 and Th1 systemic response ( Fig. 2a ). These findings were unexpected as Th1 and Th17 cells are known to play a critical role in the development of EAE. However, increasing evidence indicates that in the presence of TGF-β 1 , Th17 cells are non-pathogenic and it has been shown that TGF-β 1 inhibits T-bet expression, a transcription factor that regulates Th1/Th17-mediated autoimmunity [23] , [36] . IL-10 has been shown to protect against EAE and more importantly Th1 IFN-γ-producing cells that co-express IL-10 have been reported to display immunosuppressive properties [21] , [22] , [35] , [37] . Thus, we further investigated Th1 and Th17 responses associated with NAD + . Flow cytometry results indicated that NAD + treatment enhanced IL-10 and TGF-β by Th1 and Th17 cells, respectively ( Fig. 2a and Supplementary Fig. 2 ). As control group, CD4 + T cells were isolated from naïve mice and treated with PMA/ionomycin. As shown in Supplementary Fig. 3, naïve CD4 + T cells did not have any cytokine increase. Furthermore, granulocyte–macrophage colony-stimulating factor (GM-CSF), TGF-β 3 and IL-23 have been shown to play a critical role in Th17 pathogenicity [23] , [38] , [39] . Our results indicated that NAD + treatment reduced GM-CSF expression by CD4 + IL-17A + -producing cells, whereas IL-23R expression was increased when compared with the control group ( Fig. 2a ). However, ELISA results indicated that only TGF-β 1 was increased systemically, no differences in GM-CSF, TGF-β 3 and IL-23 were noted between the group of mice that was treated with NAD + treatment and the control group ( Supplementary Fig. 4 ). Furthermore, to assess the level of inflammation in the spinal cord, IFN-γ and IL-17A mRNA levels in the spinal cord were quantified by real-time PCR. In contrast to the control group, we could not detect IFN- γ or IL-17A mRNA in the spinal cord of NAD + -treated mice ( Fig. 2b ). These findings suggest that NAD + promotes homeostasis, despite the reduced frequency of CD4 + CD25 + Foxp3 + Tregs, by promoting immunosuppressive Th1 and Th17 cells. Therefore, we next sought to test whether NAD + protective properties were mediated in part via IL-10 production. Consistent with a previous report [35] , our results indicated that IL-10 −/− mice were very susceptible to EAE when compared with their wild-type (WT) counterparts ( Fig. 2c ). Interestingly, NAD + did not confer protection against EAE to MOG-immunized IL-10 −/− mice ( Fig. 2c ). Of note, NAD + treatment of mice did not affect the absolute number of circulating lymphocytes in the blood or spleen ( Fig. 2d ). Taken together, our results suggest that NAD + treatment alters the systemic immune response associated with EAE and induces homeostasis by inducing IL-10 and TGF-β 1 production by Th1 and Th17 cells, respectively. 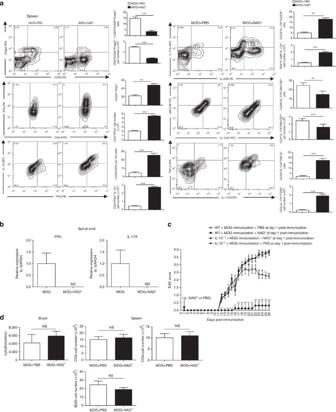Figure 2: NAD+protects against EAE through IL-10. (a) C57BL/6 mice were subjected to EAE by MOG immunization and treated daily with intraperitoneal injection of 60 mg of NAD+or a placebo solution (PBS). After 18 days, mice were euthanized and CD4+T cells were isolated from spleens, total cell number as well as frequencies of CD4+CD25+Foxp3+, CD4+IFNγ+, CD4+IFNγ+IL-10+, CD4+IL-23R+IL-17A+, CD4+IL-17A+GM-CSF+, CD4+IL-17A+TGFβ+cells were analysed by flow cytometry. (b) mRNA was extracted from the spinal cord of treated NAD+and control group animals and expression of IFN-γ and IL-17A was measured by real-time PCR. (c) Disease scores of EAE in IL-10−/−(C57BL/6 background) and wild-type (C57BL/6 background) mice treated with NAD+or a placebo solution (PBS). (d) Absolute number of lymphocytes in the blood and in the spleen (n=8–11 per group, representative plots shown). Data derived from two independent experiments; data represent mean±s.d. *P<0.05; **P<0.01; ***P<0.001; NS, not significant; ND, non-detectable. Student’st-test and Mann–WhitneyU-test were used accordingly to compare between groups. Figure 2: NAD + protects against EAE through IL-10. ( a ) C57BL/6 mice were subjected to EAE by MOG immunization and treated daily with intraperitoneal injection of 60 mg of NAD + or a placebo solution (PBS). After 18 days, mice were euthanized and CD4 + T cells were isolated from spleens, total cell number as well as frequencies of CD4 + CD25 + Foxp3 + , CD4 + IFNγ + , CD4 + IFNγ + IL-10 + , CD4 + IL-23R + IL-17A + , CD4 + IL-17A + GM-CSF + , CD4 + IL-17A + TGFβ + cells were analysed by flow cytometry. ( b ) mRNA was extracted from the spinal cord of treated NAD + and control group animals and expression of IFN-γ and IL-17A was measured by real-time PCR. ( c ) Disease scores of EAE in IL-10 −/− (C57BL/6 background) and wild-type (C57BL/6 background) mice treated with NAD + or a placebo solution (PBS). ( d ) Absolute number of lymphocytes in the blood and in the spleen ( n =8–11 per group, representative plots shown). Data derived from two independent experiments; data represent mean±s.d. * P <0.05; ** P <0.01; *** P <0.001; NS, not significant; ND, non-detectable. Student’s t -test and Mann–Whitney U -test were used accordingly to compare between groups. Full size image NAD + regulates CD4 + T-cell apoptosis and differentiation Although NAD + has been previously shown to regulate T-cell death and cytokine production [27] , [28] , [40] , [41] , [42] , its role in T-cell differentiation remains unknown. Our in vivo findings indicate that NAD + alters the systemic immune response in EAE. Therefore, we next sought to dissect the effect of NAD + on CD4 + T-cell death and differentiation in vitro under Th0, Th1, Th2, Th17 and induced regulatory T cells (iTreg) polarizing conditions. To assess the role of NAD + on CD4 + T-cell death, naïve CD4 + T cells were isolated from spleens of 5C.C7 Rag2 −/− mice, and cultured under Th0, Th1, Th2, Th17 or iTreg polarizing conditions and in the presence of increasing concentrations of NAD + . After 4 days of culture, the toxicity of NAD + was assessed by quantification of apoptotic cells using fluorochrome-labelled inhibitors of caspases (FLICA) method [43] . Our results show that treatment with NAD + of naïve CD4 + T cells in Th0 conditions resulted in a significant increase in apoptosis when compared with cells that were treated with a control solution (PBS; Fig. 3 ). These findings were consistent with a previous study that showed increased cell death of naïve CD4 + T cells in mice treated with NAD + (ref. 26 ). In contrast, CD4 + T cells that were differentiated into Th1, Th2, Th17 and iTreg were protected by NAD + against apoptosis, unlike cells that were stimulated with α-CD3/α-CD28 antibodies alone or incubated under Th0 polarizing conditions, consistent with a previous study showing that effector/memory T cells were more resistant to cell death in vivo [26] ( Fig. 3 ). 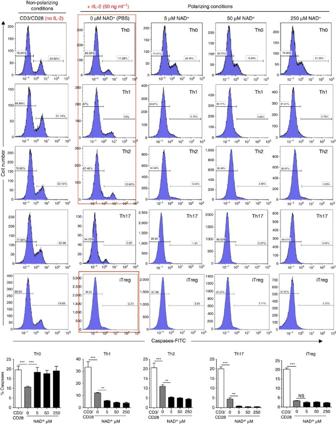Figure 3: NAD+prevents differentiating CD4+T cell from apoptosis. Sorted naïve CD4+T cells were isolated from spleens of 5C.C7Rag2−/−mice (C57BL/6 background) and activated with α-CD3/α-CD28 antibodies only or in Th0 (recombinant IL-2 cytokine at a concentration of 50 ng ml−1), Th1, Th2, Th17 or iTreg-polarizing conditions. Cells that were cultured in Th0, Th1, Th2, Th17 and iTreg polarizing conditions were stimulated with increasing concentrations of NAD+(0, 5, 50 and 250 μM). After 96 h, percentage of apoptotic cells was assessed by flow cytometry by caspase activity measurements (n=15; data derived from three independent experiments). Data represent mean±s.d. NS; not significant; **P<0.01; ***P<0.001 as determined by Student’st-test, comparing the indicated groups. Figure 3: NAD + prevents differentiating CD4 + T cell from apoptosis. Sorted naïve CD4 + T cells were isolated from spleens of 5C.C7 Rag2 −/− mice (C57BL/6 background) and activated with α-CD3/α-CD28 antibodies only or in Th0 (recombinant IL-2 cytokine at a concentration of 50 ng ml −1 ), Th1, Th2, Th17 or iTreg-polarizing conditions. Cells that were cultured in Th0, Th1, Th2, Th17 and iTreg polarizing conditions were stimulated with increasing concentrations of NAD + (0, 5, 50 and 250 μM). After 96 h, percentage of apoptotic cells was assessed by flow cytometry by caspase activity measurements ( n =15; data derived from three independent experiments). Data represent mean±s.d. NS; not significant; ** P <0.01; *** P <0.001 as determined by Student’s t -test, comparing the indicated groups. Full size image Furthermore, to determine the role of NAD + on CD4 + T-cell differentiation, cytokine profiles of 5C.C7 Rag2 −/− naïve CD4 + T cells that were cultured in Th0, Th1, Th2, Th17 and iTreg polarizing conditions were assessed by flow cytometry and ELISA. Flow cytometry analysis showed that in Th0 polarizing conditions, NAD + was able to promote a dramatic increase in CD4 + IFNγ + and a modest increase in CD4 + IL-4 + and CD4 + IL-17 + cell frequencies in a dose-dependent manner ( Fig. 4 ). However, no change in CD4 + IL-10 + cell frequencies was observed after NAD + treatment ( Fig. 4 ). In a similar manner, the increased CD4 + IFNγ + cell frequency was observed with flow cytometry sorted naïve CD4 + CD25 - CD44 low CD62L high cells from WT mice ( Supplementary Fig. 5 ). ELISA data were in line with flow cytometry results ( Supplementary Fig. 6 ). We next investigated whether NAD + regulates CD4 + T-cell differentiation under Th1 polarizing conditions. Flow cytometry analysis showed that increasing concentrations of NAD + resulted in a dramatic increase in CD4 + IFNγ + cell frequencies ( Fig. 5 ). More importantly, the results showed that NAD + was able to promote IL-10 production by IFN-γ-producing Th1 cells in sorted naïve CD4 + T cells from 5C.C7 Rag2 −/− and WT animals ( Supplementary Fig. 5 ). Of note, NAD + was able to promote a moderate increase in CD4 + IL-17 + cell frequencies ( Fig. 5 ). ELISA results were consistent with flow cytometry results ( Supplementary Fig. 6 ). 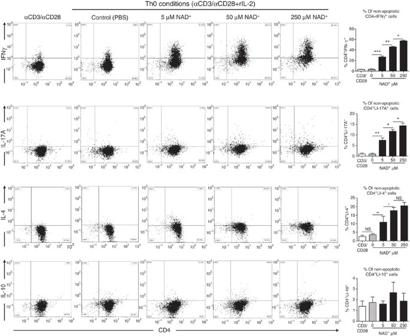Figure 4: NAD+converts naïve CD4+T cells into Th1 and Th2 as well as Th17 cells. Sorted naïve CD4+T cells were isolated from spleens of 5C.C7Rag2−/−mice (C57BL/6 background) and were activated with α-CD3/α-CD28 antibodies only or in Th0 non-polarizing conditions (with α-CD3/α-CD28 and 50 ng ml−1of recombinant IL-2 cytokine). Cells that were cultured with recombinant IL-2 were stimulated with increasing concentrations of NAD+(0, 5, 50 and 250 μM). After 96 h, percentage of CD4+IFNγ+, CD4+IL-17A+, CD4+IL-4+and CD4+IL-10+cells were assessed by flow cytometry by gating on non-apoptotic cells. To set the gates, flow cytometry dot plots were based on comparison with isotype controls, fluorescence minus one (FMO), permeabilized and unpermeabilized unstained cells (n=15; the data derived from three independent experiments). Data represent mean±s.d.; NS, not significant; *P<0.05; **P<0.01; ***P<0.001 as determined by Student’st-test, comparing the indicated groups. Figure 4: NAD + converts naïve CD4 + T cells into Th1 and Th2 as well as Th17 cells. Sorted naïve CD4 + T cells were isolated from spleens of 5C.C7 Rag2 −/− mice (C57BL/6 background) and were activated with α-CD3/α-CD28 antibodies only or in Th0 non-polarizing conditions (with α-CD3/α-CD28 and 50 ng ml −1 of recombinant IL-2 cytokine). Cells that were cultured with recombinant IL-2 were stimulated with increasing concentrations of NAD + (0, 5, 50 and 250 μM). After 96 h, percentage of CD4 + IFNγ + , CD4 + IL-17A + , CD4 + IL-4 + and CD4 + IL-10 + cells were assessed by flow cytometry by gating on non-apoptotic cells. To set the gates, flow cytometry dot plots were based on comparison with isotype controls, fluorescence minus one (FMO), permeabilized and unpermeabilized unstained cells ( n =15; the data derived from three independent experiments). Data represent mean±s.d. ; NS, not significant; * P <0.05; ** P <0.01; *** P <0.001 as determined by Student’s t -test, comparing the indicated groups. 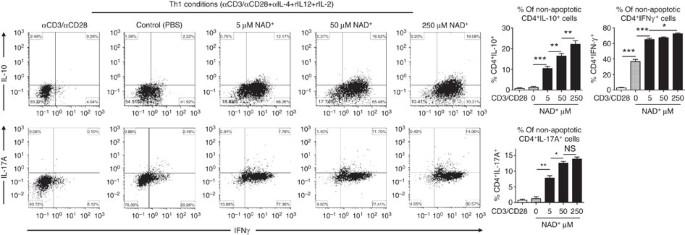Figure 5: NAD+promotes IL-10 under Th1 conditions. Sorted naïve CD4+T cells were isolated from spleens of 5C.C7Rag2−/−mice (C57BL/6 background) and were activated with α-CD3/α-CD28 antibodies only or in Th1 polarizing conditions (with α-CD3/α-CD28, 20 ng ml−1of recombinant IL-12, 50 ng ml−1of recombinant IL-2 cytokine and 10 μg ml−1of anti-IL-4). Cells in Th1 polarizing conditions were cultured in the presence of increasing concentrations of NAD+. After 96 h, percentage of CD4+IFNγ+IL-10+and CD4+IFNγ+IL-17A+cells was measured by flow cytometry by gating on non-apoptotic CD4+cells. To set the gates, flow cytometry dot plots were based on comparison with isotype controls, fluorescence minus one (FMO), permeabilized and unpermeabilized unstained cells (n=15; the data derived from three independent experiments). Data represent mean±s.d. NS, not significant *P<0.05; **P<0.01; ***P<0.001 as determined by Student’st-test, comparing the indicated groups. Full size image Figure 5: NAD + promotes IL-10 under Th1 conditions. Sorted naïve CD4 + T cells were isolated from spleens of 5C.C7 Rag2 −/− mice (C57BL/6 background) and were activated with α-CD3/α-CD28 antibodies only or in Th1 polarizing conditions (with α-CD3/α-CD28, 20 ng ml −1 of recombinant IL-12, 50 ng ml −1 of recombinant IL-2 cytokine and 10 μg ml −1 of anti-IL-4). Cells in Th1 polarizing conditions were cultured in the presence of increasing concentrations of NAD + . After 96 h, percentage of CD4 + IFNγ + IL-10 + and CD4 + IFNγ + IL-17A + cells was measured by flow cytometry by gating on non-apoptotic CD4 + cells. To set the gates, flow cytometry dot plots were based on comparison with isotype controls, fluorescence minus one (FMO), permeabilized and unpermeabilized unstained cells ( n =15; the data derived from three independent experiments). Data represent mean±s.d. NS, not significant * P <0.05; ** P <0.01; *** P <0.001 as determined by Student’s t -test, comparing the indicated groups. Full size image Under Th2 polarizing conditions, cultured naïve CD4 + T cells from 5C.C7 Rag2 −/− mice in the presence of NAD + resulted in a strong increase in CD4 + IL-4 + IL-10 + and a modest increase in CD4 + IL-4 + IL-17A + cell frequency ( Fig. 6 ), consistent with IL-10 and IL-17A secretion levels ( Supplementary Fig. 6 ). Of note, increased cell frequency of CD4 + IL-4 + IL-10 + was observed with naïve WT CD4 + cells as well ( Supplementary Fig. 5 ). Under Th17 polarizing conditions, addition of NAD + did not alter T-cell differentiation ( Supplementary Fig. 7 ) and cytokine production levels ( Supplementary Fig. 6 ). In contrast, under iTreg polarizing conditions, fluorescence-activated cell sorting analysis revealed a robust increase in the frequency of CD4 + TGFβ + IL-17A + in naïve CD4 + T cells from both 5C.C7 Rag2 −/− ( Supplementary Fig. 8 ) and WT mice ( Supplementary Fig. 5 ). However, we found no changes in the frequency of CD4 + IL-10 + IL-17A + cells. ELISA findings were consistent with flow cytometry ( Supplementary Fig. 6 ). 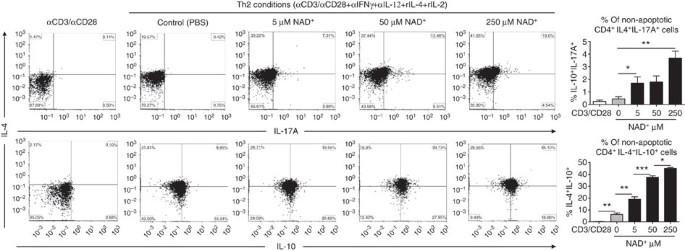Figure 6: NAD+promotes IL-10 and IL-17A in Th2 polarizing conditions. Sorted naïve CD4+T cells were isolated from spleens of 5C.C7Rag2−/−mice (C57BL/6 background) and were activated with α-CD3/α-CD28 antibodies only or in Th2 polarizing conditions (with α-CD3/α-CD28, 20 ng ml−1of recombinant IL-4, 50 ng ml−1of recombinant IL-2, 10 μg ml−1of anti-IL-12 and anti-IFN-γ antibodies). Cells in Th2 polarizing conditions were cultured in the presence of increasing concentrations of NAD+. After 96 h, percentage of CD4+IL-4+IL-10+and CD4+IL-4+IL-17A+cells was measured by flow cytometry by gating on non-apoptotic CD4+cells. To set the gates, flow cytometry dot plots were based on comparison with isotype controls, fluorescence minus one (FMO), permeabilized and unpermeabilized unstained cells (n=15; the data derived from three independent experiments). Data represent mean±s.d. NS, not significant. *P<0.05; **P<0.01; ***P<0.001 as determined by Student’st-test, comparing the indicated groups. Figure 6: NAD + promotes IL-10 and IL-17A in Th2 polarizing conditions. Sorted naïve CD4 + T cells were isolated from spleens of 5C.C7 Rag2 −/− mice (C57BL/6 background) and were activated with α-CD3/α-CD28 antibodies only or in Th2 polarizing conditions (with α-CD3/α-CD28, 20 ng ml −1 of recombinant IL-4, 50 ng ml −1 of recombinant IL-2, 10 μg ml −1 of anti-IL-12 and anti-IFN-γ antibodies). Cells in Th2 polarizing conditions were cultured in the presence of increasing concentrations of NAD + . After 96 h, percentage of CD4 + IL-4 + IL-10 + and CD4 + IL-4 + IL-17A + cells was measured by flow cytometry by gating on non-apoptotic CD4 + cells. To set the gates, flow cytometry dot plots were based on comparison with isotype controls, fluorescence minus one (FMO), permeabilized and unpermeabilized unstained cells ( n =15; the data derived from three independent experiments). Data represent mean±s.d. NS, not significant. * P <0.05; ** P <0.01; *** P <0.001 as determined by Student’s t -test, comparing the indicated groups. Full size image Although our data indicate that NAD + plays an important role in naïve CD4 + T-cell differentiation/apoptosis, it is however unclear how NAD + can protect against EAE 15 days after MOG immunization when CD4 + T cells have already polarized into a specific Th phenotype. Thus, we next investigated the impact of NAD + on differentiated CD4 + T cells. Naïve CD4 + CD25 − CD44 low CD62L high T cells were cultured (0.5 × 10 6 cells) in Th1 or Th2 polarizing conditions. After 1 week, polarized Th1 and Th2 CD4 + T cells were incubated in the presence of NAD + during 72 h, rested and re-incubated in Th1 or Th2 polarizing conditions ( Fig. 7a,b ). Cell number counts indicated that after 1 week naïve CD4 + T cells proliferated from 0.5 × 10 6 to 2 × 10 6 and 3.5 × 10 6 cells in Th1 and Th2 polarizing conditions, respectively ( Fig. 7a,b ). More importantly, when incubated in the presence of NAD + for only 72 h, Th1 and Th2 polarized cells proliferated dramatically and the number of Th1 (2 × 10 6 cells) and Th2 (3.5 × 10 6 cells) CD4 + cells increased significantly (>6 × 10 6 for Th1 cells and >8 × 10 6 for Th2 cells). Although NAD + promoted Th1 and Th2 cell proliferation, flow cytometry analysis ( Fig. 7a,b ) indicated that NAD + reduced dramatically Th1 (IFN-γ) and Th2 (IL-4 and IL-10) cytokine expression levels as shown by frequency and total number of cells. To further assess how NAD + altered CD4 + T-cell differentiation, Th1 and Th2 cultured in the presence of NAD + were rested in media for 72 h and re-stimulated in Th1 or Th2 polarizing conditions. After 10 days of culture, only 35% of CD4 + T cells were able to produce IFN-γ after Th1 re-stimulation ( Fig. 7a ). Similarly, upon Th2 re-stimulation only 20% of CD4 + T cells were able to produce IL-10. More importantly, CD4 + T cells were not able to produce IL-4 even 10 days after Th2 re-stimulation ( Fig. 7b ). Of note, after only 1 week and in similar Th1 or Th2 polarizing conditions, more than 90% of CD4 + T cells were IFNγ + or IL4 + IL10 + , respectively. Collectively, these results demonstrate that NAD + alters CD4 + T-cell apoptosis/proliferation and differentiation in polarized CD4 + T cells and suggest that NAD + may reverse the diseases progression by altering differentiated CD4 + T cells. Moreover, the fact that NAD + induces a robust cytokine production in naïve CD4 + T cells but blocks cytokine production in differentiated cells suggests that NAD + regulates CD4 + T-cell differentiation through an alternative pathway that is distinct from the classical cytokine pathway [4] , [16] , [44] , [45] , [46] , [47] . 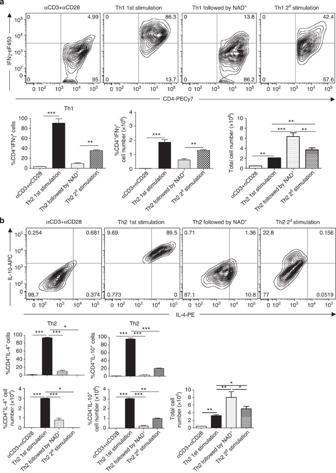Figure 7: NAD+does not induce cell death. Sorted naïve CD4+T cells were isolated from spleens of wild-type C57BL/6 mice and cultured (0.5 × 106cells per well) in Th1 (with α-CD3/α-CD28, 50 ng ml−1of recombinant IL-12, 50 ng ml−1of recombinant IL-2 cytokine and 10 μg ml−1of anti-IL-4;a) and Th2 (with α-CD3/α-CD28, 50 ng ml−1of recombinant IL-4, 50 ng ml−1of recombinant IL-2, 10 μg ml−1of anti-IL-12 and anti-IFN-γ antibodies;b) polarizing conditions for 1 week, washed and followed by and incubation period of 72 h with NAD+(100 μM). Cells were then rested for 72 h and a 2dTh1 or Th2 stimulation was performed. After 10 days, total cell numbers and frequencies of CD4+IFNγ+and CD4+IL-4+IL-10+cells were measured by flow cytometry by gaiting on CD4+T cells; cell proliferation was assessed by cell counting after each incubation period (n=10; the data derived from two independent experiments). Data represent mean±s.d. NS, not significant. *P<0.05; **P<0.01; ***P<0.001 as determined by Student’st-test, comparing the indicated groups. Figure 7: NAD + does not induce cell death. Sorted naïve CD4 + T cells were isolated from spleens of wild-type C57BL/6 mice and cultured (0.5 × 10 6 cells per well) in Th1 (with α-CD3/α-CD28, 50 ng ml −1 of recombinant IL-12, 50 ng ml −1 of recombinant IL-2 cytokine and 10 μg ml −1 of anti-IL-4; a ) and Th2 (with α-CD3/α-CD28, 50 ng ml −1 of recombinant IL-4, 50 ng ml −1 of recombinant IL-2, 10 μg ml −1 of anti-IL-12 and anti-IFN-γ antibodies; b ) polarizing conditions for 1 week, washed and followed by and incubation period of 72 h with NAD + (100 μM). Cells were then rested for 72 h and a 2 d Th1 or Th2 stimulation was performed. After 10 days, total cell numbers and frequencies of CD4 + IFNγ + and CD4 + IL-4 + IL-10 + cells were measured by flow cytometry by gaiting on CD4 + T cells; cell proliferation was assessed by cell counting after each incubation period ( n =10; the data derived from two independent experiments). Data represent mean±s.d. NS, not significant. * P <0.05; ** P <0.01; *** P <0.001 as determined by Student’s t -test, comparing the indicated groups. Full size image NAD + signals and protects against EAE via Tph1 Our findings clearly demonstrate that NAD + is able to alter CD4 + T-cell differentiation in vitro and in vivo . More importantly, in vitro results indicated that NAD + is able to override Th1, Th2 and iTreg, but not Th17 polarizing conditions. Therefore, we sought to profile NAD + -induced perturbations in gene expression profile of Th0, Th1, Th2 and iTreg polarized cells. Although increasing concentrations of NAD + promoted IFN-γ-producing cells in a dose-dependent manner in Th0 and Th1 polarizing conditions, the results indicated that gene expression of T-bet , the master regulator of Th1 development [44] , [47] , was reduced ( Supplementary Fig. 9 ). Of note, no changes in the expression level of master regulators of Th2 ( GATA3 , STAT5a , STAT6 ) or Th17 ( ROR γ t ) were observed under Th0 polarizing conditions ( Supplementary Fig. 9 ). Furthermore, a dramatic decrease (>10-fold) in expression of GATA3 , a transcription factor that regulates Th2 cell differentiation, occurred under Th2 polarizing conditions. More importantly, in the presence of NAD + , Foxp3 , the master regulator of Tregs development was not detected under iTreg polarizing conditions ( Supplementary Fig. 9 ). Collectively, these findings suggest that NAD + inhibits the expression of well-established master regulators of CD4 + T-cell development and may induce CD4 + T-cell differentiation through an alternative, unconventional pathway. Therefore, to identify potential molecules involved in NAD + -mediated CD4 + T-cell regulation, genome-wide gene expression profiles were assessed by microarray analysis. Interestingly, Tph1 , a gene encoding for an enzyme that is mostly described as a mast cell product [48] , was found among the top 20 upregulated genes in Th0, Th1, Th2 and iTreg-polarized cells ( Supplementary Fig. 10a ). Tph1 upregulation was confirmed by real-time PCR in naïve CD4 + T cells isolated from both, WT and 5C.C7 Rag2 −/− mice ( Supplementary Fig. 10b ). Similar to naïve CD4 + T cells that were cultured under Th0, Th1, Th2 and iTreg polarizing conditions with NAD + , polarized Th1 and Th2 CD4 + T cells had a decreased mRNA levels of T-bet and GATA3 , whereas Tph1 was dramatically increased ( Supplementary Fig. 11 ). Although ROR γ t expression was reduced in Th17 polarizing conditions in the presence of 50 and 250 μM of NAD + , the decrease was significant only for the latter concentration ( Supplementary Fig. 9 ). Furthermore, Ingenuity Pathway Analysis predicted significant perturbations by NAD + of other pathways involved in T-cell differentiation, IL-17 and IL-10 signalling ( Supplementary Table 1 ). Because Tph1 has recently been reported to prevent allograft rejection and EAE [48] , we interrogated its involvement in vivo in mediating the protection from EAE and regulation of CD4 + T-cell differentiation by NAD + . Mice were subjected to EAE and were treated daily with PBS or NAD + . Half of the animals in each group also received p -chlorophenylalanine, a specific inhibitor of Tph1. Onset of clinical signs of EAE in mice immunized with MOG peptide and treated with a placebo solution appeared after 11 days ( Fig. 8a ). Similar to the results described above ( Fig. 1a and Supplementary Movie 1d and f ), mice treated with NAD + were protected from EAE ( Fig. 8a ). However, when NAD + -treated mice were administered the Tph1 inhibitor, onset of clinical signs of EAE appeared after 12 days ( Fig. 8a ). Furthermore, on day 12 after MOG immunization, mice treated with NAD + and p -chlorophenylalanine exhibited more severe clinical signs of EAE than did immunized mice that were treated with a placebo solution ( Fig. 8a ). Mice treated with Tph1 inhibitor exhibited hindlimb paralysis and became rapidly lethargic. Flow cytometry showed that the combination of NAD + treatment with Tph1 inhibition caused a systemic reduction in the number of CD4 + IL-17A + and CD4 + IL-10 + IFNγ + and CD4 + CD25 + Foxp3 + cells ( Fig. 8b ). Collectively, these results indicate that Tph1 plays a critical role in NAD + protective properties against EAE and CD4 + T helper cell and differentiation. 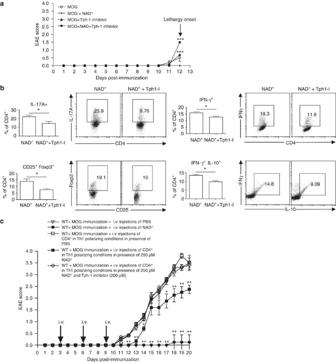Figure 8: NAD+regulates CD4+T-cell differentiation throughTph1. (a) Behavioural scores of EAE in wild-type C57BL/6 mice treated either with intraperitoneal injection of 60 mg of NAD+or a placebo solution (PBS). An additional group of mice was treated with intraperitoneal injections of NAD+and p-chlorophenylalanin (Tph1 inhibitor). As a control group, wild-type mice were treated with Tph1 inhibitor alone (n=5 per group). (b) CD4+T cells were isolated from spleens 13 days after EAE induction and CD4+frequencies of CD25+Foxp3+, IL-17A+, IFNγ+and IFNγ+IL-10+cells were analysed by flow cytometry. (c) Behavioural scores of EAE in wild-type mice (C57BL/6 background) treated at days 3, 6 and 9 with intravenous injections of sorted naïve CD4+CD25+CD44lowCD62LhighT cells (2 × 106cells) that were cultured during 4 days in Th1 polarizing conditions in the presence of NAD+(250 μM) or a placebo solution (PBS). As control groups, wild-type mice were subjected to EAE and treated with NAD+(60 mg) or PBS intravenously at days 3, 6 and 9 (n=8–11 per group). Data derived from two independent experiments; data represent mean±s.d. *P<0.05; **P<0.01; ***P<0.001 significant as determined by Student’st-test and Mann–WhitneyU-test were used accordingly to compare between groups. i.p., intraperitoneal; i.v. intravenous. Figure 8: NAD + regulates CD4 + T-cell differentiation through Tph1 . ( a ) Behavioural scores of EAE in wild-type C57BL/6 mice treated either with intraperitoneal injection of 60 mg of NAD + or a placebo solution (PBS). An additional group of mice was treated with intraperitoneal injections of NAD + and p-chlorophenylalanin (Tph1 inhibitor). As a control group, wild-type mice were treated with Tph1 inhibitor alone ( n =5 per group). ( b ) CD4 + T cells were isolated from spleens 13 days after EAE induction and CD4 + frequencies of CD25 + Foxp3 + , IL-17A + , IFNγ + and IFNγ + IL-10 + cells were analysed by flow cytometry. ( c ) Behavioural scores of EAE in wild-type mice (C57BL/6 background) treated at days 3, 6 and 9 with intravenous injections of sorted naïve CD4 + CD25 + CD44 low CD62L high T cells (2 × 10 6 cells) that were cultured during 4 days in Th1 polarizing conditions in the presence of NAD + (250 μM) or a placebo solution (PBS). As control groups, wild-type mice were subjected to EAE and treated with NAD + (60 mg) or PBS intravenously at days 3, 6 and 9 ( n =8–11 per group). Data derived from two independent experiments; data represent mean±s.d. * P <0.05; ** P <0.01; *** P <0.001 significant as determined by Student’s t -test and Mann–Whitney U -test were used accordingly to compare between groups. i.p., intraperitoneal; i.v. intravenous. Full size image NAD + protects against EAE through IL-10 and Tr1 cells It is well established that Th1 IL-10-producing cells are robust immunosuppressive cells that promote homeostasis [20] , [22] , [37] and we found that NAD + induces IL-10 production by Th1 cells in vitro and in vivo . Thus, to investigate whether NAD + protective properties were mediated through IL-10 production by Th1 cells, naïve CD4 + CD25 − CD44 low CD62L high T cells were obtained by cell sorting and cultured during 4 days in Th1 polarizing conditions in the presence of NAD + (250 μM) or vehicle (PBS) and used in an adoptive transfer experiment. After 4 days of culture, cells were collected and injected intravenously (2 × 10 6 cells per injection) at days 3, 6 and 9 in WT mice that were subjected to EAE. Similar to our previous results, mice treated with NAD + were protected against EAE, whereas mice treated with PBS and mice that received CD4 + T cells that were cultured in the presence of a placebo solution did develop severe EAE with clinical onset at day 11 ( Fig. 8c ). In contrast, mice that received CD4 + T cells that were cultured in the presence of NAD + had a significant delayed clinical onset (day 13) and developed a less severe EAE than the control groups ( Fig. 8c ). In addition, our data indicate that NAD + promotes IL-10 production by Th1 cells through Tph1. Thus, to assess the role of Tph1 in IL-10 production by Th1 cells and its role in NAD + mediated protective properties, an additional group of mice received intravenous injections of CD4 + T cells that were previously cultured with NAD + (250 μM) and Tph1 inhibitor (200 μM). Similar to mice that received CD4 + T cells that were cultured in the presence of a placebo solution did develop severe EAE with clinical onset at day 11 ( Fig. 8c ). Taken together, these results indicate that NAD + protective properties are mediated via IL-10- and Th1-IL-10-producing cells and that Tph1 signalling pathway plays an important role. NAD + enhances IFN-γ production independently of T-bet Our previous results indicated that NAD + overrides the cytokine environment and alters CD4 + T-cell differentiation. Our findings indicate that in Th0 polarizing conditions NAD + was able to promote IFN-γ production. In addition, we have shown that NAD + inhibits cytokine production of polarized Th1 and Th2 CD4 + T cells and inhibits the expression of several major transcription factors that have been shown to play a central role in CD4 + T-cell differentiation such as T-bet , GATA3 and Foxp3 (refs 44 , 45 , 49 ). In contrast, microarray analysis and real-time PCR results showed an increased Tph1 mRNA levels suggesting that NAD + regulates CD4 + T-cell differentiation through Tph1 and more importantly independently of well-established transcription factors. Thus, we next investigated whether NAD + was able to regulate CD4 + T-cell differentiation and promote cytokine production in the absence of major transcription factors. Naïve CD4 + CD25 − CD44 low CD62L high T cells were isolated from WT and T-bet −/− mice and cultured in Th1 polarizing condition in the presence of NAD + or a placebo solution (PBS). After 1 week, cells were analysed by flow cytometry. As shown in Fig. 9 , NAD + induced a very robust IFN-γ production by WT naïve CD4 + T cells (~73%) cultured in Th1 polarizing conditions when compared with the control group of WT naïve CD4 + T cells that were cultured in Th1 polarizing conditions and PBS (~25%). Furthermore, NAD + treatment of naïve CD4 + T cells isolated from T-bet −/− mice resulted in a dramatic increase of CD4 + IFNγ + cells (~58%) when compared with Th1 polarizing conditions (~8%). More importantly, ~58% of T-bet −/− CD4 + T cells were able to produce IFN-γ, whereas only ~25% of WT CD4 + T cells were able to produce IFNγ in Th1 polarizing conditions ( Fig. 9 ). Taken together, these results demonstrate that NAD + is a robust IFN-γ inducer and more importantly that NAD + regulates cytokine production independently of the classical transcription factors. 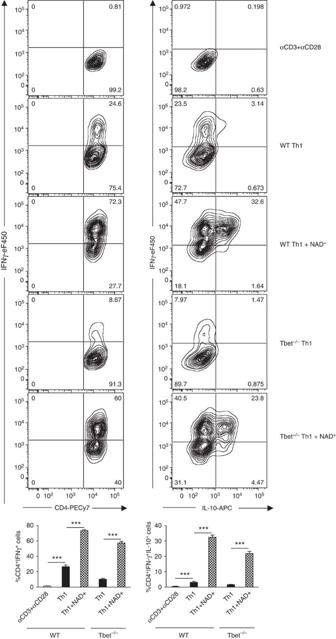Figure 9: NAD+promotes IFN-γ independently of the master regulatorT-bet. Naïve CD4+T cells were isolated from wild-type andT-bet−/−mice (C57Bl/6 background) and cultured in Th1 polarizing condition (with α-CD3/α-CD28, 50 ng ml−1of recombinant IL-12, 50 ng ml−1of recombinant IL-2 cytokine and 10 μg ml−1of anti-IL-4) in the presence of NAD+or a placebo solution (PBS). After 1 week, CD4+IFNγ+and CD4+IFNγ+IL-10+cells were measured by flow cytometry by gating on CD4+T cells (n=10; the data derived from two independent experiments). Data represent mean±s.d. NS, not significant. ***P<0.001 as determined by Student’st-test, comparing the indicated groups. Figure 9: NAD + promotes IFN-γ independently of the master regulator T-bet . Naïve CD4 + T cells were isolated from wild-type and T-bet −/− mice (C57Bl/6 background) and cultured in Th1 polarizing condition (with α-CD3/α-CD28, 50 ng ml −1 of recombinant IL-12, 50 ng ml −1 of recombinant IL-2 cytokine and 10 μg ml −1 of anti-IL-4) in the presence of NAD + or a placebo solution (PBS). After 1 week, CD4 + IFNγ + and CD4 + IFNγ + IL-10 + cells were measured by flow cytometry by gating on CD4 + T cells ( n =10; the data derived from two independent experiments). Data represent mean±s.d. NS, not significant. *** P <0.001 as determined by Student’s t -test, comparing the indicated groups. Full size image In the present work, we report that NAD + is able to regulate CD4 + T-cell differentiation ( Fig. 10 ). In addition, our data indicate that NAD + promotes a robust systemic IL-10 and TGF-β 1 production by Th1 and Th17 cells, respectively. IL-10 and TGF-β 1 are two prominent immunosuppressive cytokines that were shown to protect from EAE [35] . The central role of IL-10 in NAD + -mediated protection against EAE was demonstrated when IL-10 −/− mice treated with NAD + and subjected to EAE developed severe clinical symptoms. More importantly, Th1 cells that co-express IL-10 have been shown to have immunosuppressive properties and to prevent from exaggerated immune responses and concomitant tissue damage. Because of their anti-inflammatory properties, IL-10-producing Th1 cells were termed Tr1 cells [22] . Here we show that adoptive transfer of CD4 + T cells that were differentiated in vitro under Th1 polarizing conditions in the presence of NAD + significantly delayed the clinical onset and reduced the severity of the disease. These findings are in line with previous studies that have shown that IL-10 production by IFN-γ-producing Th1 cells can prevent tissue damage and autoimmune diseases [21] , [37] . Nevertheless, mice that received CD4 + T cells that were differentiated in vitro under Th1 polarizing conditions in the presence of NAD + still developed mild EAE. A recent study showed that in the presence of TGF-β 1 , Th17 cells are non-pathogenic [23] and it is well known that TGF-β 1 is a robust immunosuppressive cytokine [50] . Thus, we cannot rule out that the increased level of TGF-β 1 by Th17 cells following NAD + treatment may attenuate Th17 pathogenicity and/or promote homeostasis. In addition, IL-23, TGF-β 3 and GM-CSF have been shown to play a critical role in Th17 pathogenicity and EAE [23] , [38] . In our study, we could not detect differences in IL-23, TGF-β 3 and GM-CSF systemic levels between the NAD + -treated mice and the control group. Although flow cytometry analysis showed that NAD + treatment resulted in a modest decrease of GM-CSF production by CD4 + IL-17A + cells and an increased expression of IL-23R, we do not believe that IL-23, TGF-β 3 or GM-CSF play a role in NAD + signalling machinery. 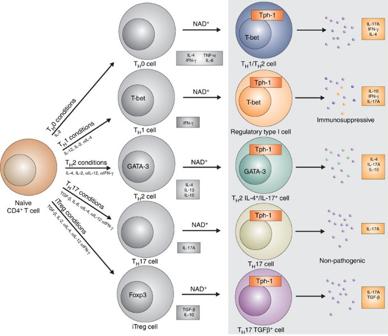Figure 10: NAD+a master regulator of CD4+ T-cell differentiation. After T-cell antigen receptor (TCR) engagement, NAD+promotes naïve CD4+T cell into Th1, Th2 and Th17 cells. NAD+promotes the conversion of Th1-IFN-γ-producing cells into regulatory type 1 cells that co-produce IFN-γ and IL-10 with immunosuppressive properties. NAD+promotes IL-10 and IL-17A cytokines by Th2 cells. NAD+does not affect Th17 cytokine conditions but drives the switch of iTreg into Th17 TGF-β-producing cells. NAD+regulates CD4+T-cell differentiation throughTph1. Figure 10: NAD + a master regulator of CD4+ T-cell differentiation. After T-cell antigen receptor (TCR) engagement, NAD + promotes naïve CD4 + T cell into Th1, Th2 and Th17 cells. NAD + promotes the conversion of Th1-IFN-γ-producing cells into regulatory type 1 cells that co-produce IFN-γ and IL-10 with immunosuppressive properties. NAD + promotes IL-10 and IL-17A cytokines by Th2 cells. NAD + does not affect Th17 cytokine conditions but drives the switch of iTreg into Th17 TGF-β-producing cells. NAD + regulates CD4 + T-cell differentiation through Tph1 . Full size image T-bet has been shown to play a critical role in controlling Th1/Th17-mediated autoimmunity [12] . T-bet -deficient mice have been shown to be resistant to autoimmunity, whereas IFN-γ-, IFN-γ receptor- and IL-17-deficient mice remain susceptible to EAE [12] . Our study demonstrates that NAD + reduces the expression level of T-bet under Th0, Th1 polarizing conditions and in differentiated Th1 cells, suggesting that NAD + may protect against EAE by inhibiting T-bet expression and thus altering Th1/Th17-mediated autoimmunity. Bruzzone et al. have shown that depletion of NAD + using FK866, an inhibitor of a key enzyme for NAD + biosynthesis, reduced clinical symptoms in EAE. The study showed that NAD + depletion with FK866 spared resting T lymphocytes and targeted specifically activated T lymphocytes resulting in increased apoptosis, reduced proliferation and cytokine production [25] . In contrast, in our study, we showed that treatment with NAD + -protected activated CD4 + T cells from apoptosis and instead regulated their differentiation. Thus, we believe that NAD + depletion by FK866 reduced EAE clinical symptoms mainly by inducing cell death of activated cells, whereas treatment with NAD + protected against EAE by inducing homeostasis and by promoting myelin regeneration and neuroregeneration. Furthermore, NAD + was able not only to block but also to reverse EAE progression by restoring myelin and favouring axonal regeneration, suggesting that NAD + may promote this process by inhibiting the inflammatory response or might act directly on other pathways involved in the CNS in particular in maintaining pluripotency [30] . Initially, NAD + was used as a therapeutic agent to treat schizophrenic patients [51] , [52] . Although a more recent study suggested that NAD + might prevent from axonal degeneration [24] , the direct impact of NAD + on the CNS remains unclear and warrants further investigation. Of note, low dose of NAD + such as 10 mg was effective in protecting against EAE. According to many reports and the Food and Drug Administration [53] guidelines, injection of 10 mg in our animal model corresponds to a dose of 1.6 g for an individual of 70 kg, which is a reasonable daily dose for patients. Moreover, our study has uncovered a new role of NAD + in CD4 + T-cell differentiation. Under Th1 polarizing conditions and in the presence of NAD + , CD4 + T helper cells were able to rapidly secrete high amounts of IL-10, conventionally considered as a Th2 cytokine. Interestingly, previous studies have shown that Th1 cells are able to produce IL-10 in culture when provided longer incubation time (2–5 weeks) and high T-cell antigen receptor stimulation [54] or chronic Th1 activation [20] . In our hands, NAD + was able to induce IL-10 secretion by IFN-γ-producing Th1 cells within hours without high T-cell antigen receptor stimulation, indicating that NAD + is a robust inducer. Although it is well accepted that IL-4 inhibits IL-17A production under Th2 polarizing conditions [5] , [7] , [15] , Wang et al. have described a CD4 + Th2 subset that co-produces IL-4 and IL-17A and have shown that these cells were the main cause of lung inflammation in the chronic stage of asthma [55] . However, the mechanisms that promote CD4 + IL-4 + IL-17A + cell development remain unknown. The mechanism of action of NAD + was confirmed, in vitro , with its capacity to convert iTregs into Th17 cells even in the presence of IL-2, a cytokine that is known to prevent Th17 lineage commitment [56] , [57] . More importantly, T-bet and GATA3 , two transcription factors that regulate CD4 + T cell Th1/Th2 fate decision were downregulated by NAD + , whereas Foxp3 , the master regulator of Tregs, was not detected, suggesting that NAD + regulates CD4 + T-cell differentiation through an alternative pathway. This alternative pathway was demonstrated using naïve T-bet −/− CD4 + T cells. In the presence of NAD + , ~58% of T-bet −/− CD4 + T cells were able to produce IFN-γ, whereas only ~8% were able to produce IFN-γ in solely Th1 polarizing conditions. More importantly, only 25% of WT CD4 + T cells were IFN-γ in Th1 polarizing conditions, indicating that NAD + not only promotes IFN-γ production independently of T-bet but also underscoring NAD + as a more potent IFN-γ inducer than Th1 polarizing conditions. In parallel to the decreased expression of T-bet , GATA3 and Foxp3 , NAD + induced a robust increase in Tph1 expression by CD4 + T helper cells under Th polarizing conditions, suggesting a central role in NAD + -mediated CD4 + T-cell differentiation. Indeed, treatment with a Tph1 inhibitor dampened the systemic IL-17A and IL-10/IFN-γ responses observed after NAD + administration, confirming that Tph1 is critical in NAD + -mediated T-cell differentiation. Moreover, mice treated with NAD + and Tph1 inhibitor simultaneously developed a more severe EAE than mice that were subjected to MOG immunization and treated with a placebo solution, indicating that Tph1 signalling pathway plays a critical role in NAD + protective properties against EAE. These findings were in line with a previous study that showed that Tph1-deficient mice were more susceptible to EAE [48] . In addition, the combination of NAD + and Tph1 inhibitor developed severe lethargy 13 days following MOG immunization and animals had to be euthanized. The cause of death was not due to MOG immunization but was most likely the result of heart failure and breathing difficulties. Indeed, Tph1 inhibition has been shown to promote serotonin depletion, a crucial neurotransmitter [58] , causing breathing difficulties and inducing heart failure [59] . In conclusion, our study underscores NAD + as a major regulator of CD4 + T-cell differentiation that signals through a novel pathway that is distinct from the classical pathway described almost three decades ago [2] , [3] , [4] . Furthermore, our study demonstrates that NAD + acts independently of the major transcription factors described [16] , [44] , [45] , [46] , [47] , [49] and signals through Tph1 enzymatic pathway. On a clinical aspect, our study unravels the therapeutic potential of NAD + as a homeostatic agent in a myriad of diseases. The unique property of NAD + in inducing homeostasis that is not mediated by CD4 + CD25 + Foxp3 + regulatory T cells may benefit immunodeficient patients that result from mutations in the Foxp3 gene [60] . In addition to its antitumour properties [27] , NAD + may be the ideal molecule to treat autoimmune diseases such as MS, type 1 diabetes and inflammatory bowel disease in which IL-10 has been shown to play a central role [61] . Moreover, NAD + homeostatic properties could be used as therapy beyond autoimmune diseases, including acute and chronic inflammatory diseases [62] . Animals Eight- to ten-week old female B10.A-Rag2tm1FwaH2-T18aTg or wild-type (WT) mice on a C57BL/6 background were purchased from Taconic. B6.129P2-IL10 tm1Cgn /J and B6.129S6- Tbx21 tm1Glm /J mice were purchased from the Jackson Laboratory. Animal use and care were in accordance with the National Institutes of Health and Institutional Animal Care and Use Committee guidelines. Cell isolation Single-cell leukocyte suspensions were obtained from spleens of 5- to 10-week-old 5C.C7 Rag2 −/− , T-bet −/− or WT mice. Depletion of non-CD4 + T cells was done using biotin-conjugated monoclonal anti-mouse antibodies against CD8α, CD11b, CD45R, CD49b, Ter-119 and anti-biotin magnetic beads (Miltenyi Biotec). Cells were further sorted using α-CD4-PE and α-PE magnetic beads (Miltenyi Biotec) and CD4+CD25-CD44lowCD62Lhigh (all eBioscience) cells were sorted by flow cytometry. All antibodies were used at a concentration of 1–2 μg per 1 × 10 6 cells. Purities of CD4 + CD25 - CD44 low CD62L high T cells after isolation were >99.2%. Cell culture Isolated CD4 + T cells were cultured in 24-well flat bottom plates (0.5 × 10 6 cells per well) in 0.5 ml of complete RPMI 1640 media (supplemented with 10% FCS, 200 mM L -glutamine, 100 U ml −1 penicillin/streptomycin and 5 × 10 -5 M 2-mercaptoethanol (RP-10) in the presence of 10 μg ml −1 plate-bound anti-mouse α-CD3 (17A2) and 2 μg ml −1 soluble α-CD28 (37.51) in addition to 50 ng ml −1 recombinant mouse IL-2 (all eBioscience). NAD + (Sigma-Aldrich) was diluted in PBS and added as indicated. Cells were cultured in polarizing Th1 (50 ng ml −1 of recombinant IL-12 and 10 μg ml −1 of anti-IL-4), Th2 (50 ng ml −1 of recombinant IL-4, 10 μg ml −1 of anti-IFN-γ), Th17 (10 ng ml −1 of recombinant TGF-β, 100 ng ml −1 of recombinant IL-6, 10 μg ml −1 of anti-IFN-γ and 10 μg ml −1 of anti-IL4) or iTreg (10 ng ml −1 of recombinant TGF-β, 10 μg ml −1 of anti-IFN-γ and 10 μg ml −1 of anti-IL4) conditions. All recombinant cytokines and antibodies were purchased from eBioscience except recombinant TGF-β cytokine (R&D Systems). After 96 h of culture supernatants and cells were collected and analysed by ELISA and flow cytometry, respectively. To investigate the impact of NAD + on polarized CD4 + T cells, naïve CD4 + T cells were isolated and cultured in Th1 or Th2 polarizing conditions as described above. After 1 week, cells were washed and incubated in the presence of NAD + (100 μM) or PBS. After 72 h, cells were rested during an additional 72 h and re-stimulated with Th1 or Th2 polarizing conditions. After 10 days, cells were stained and analysed by flow cytometry. Flow cytometry Fluorescence-labelled anti-mouse α-CD4 (GK1.5), α-CD25 (PC61), α-IFN-γ (XMG1.2) and unlabelled α-CD16/CD32 (2.4G2) antibodies were obtained from BD Biosciences. Fluorescence-labelled anti-mouse α-IL-4 (FJK-16s), α-IL-10 (JES5-16E3), α-IL-17A (eBio17B7), anti-GM-CSF (MP1-22E9), anti-Foxp3 (FJK-16s) and anti-TGFβ 1 (TW7-16B4) were obtained from eBioscience. Anti-mouse anti-IL23R (753317) was purchased from R&D systems. All antibodies were used at a concentration of 2–5 μg per 1 × 10 6 cells. To set the gates, flow cytometry dot plots were based on comparison with isotype controls, fluorescence minus one, permeabilized and unpermeabilized unstained cells. Intracellular staining for IL-4, IL-10, IL-17A, IFN-γ, GM-CSF and TGF-β was performed according to the manufacturers’ protocols. Splenocytes were re-stimulated in complete media (RPMI media containing 10% FCS, 1% L -glutamine, 1% penicillin/streptomycin; all from Bio Whittaker) for 4 h at 37 °C with ionomycin, phorbol 12-myristate 13-acetate and Brefeldin A (eBioscience). Cells were fixed and permeabilized using Cytofix/Cytoperm solution (BD Biosciences). Flow cytometry measurements of single-cell suspensions for in vivo experiments were performed on a FACSCalibur using standard procedures and data were analysed using FlowJo software (Tree Star). Flow cytometry measurements for in vitro experiments were performed on MoFlo Astrios (Beckman Coulter) and data were analysed using Kaluza software (Beckman Coulter). Apoptosis Apoptosis was assessed by caspase (caspase-1, -3, -4, -5, -6, -7, -8 and -9) activity measurements. Caspases activities were determined by flow cytometry using FAM-fluorochrome inhibitor of caspases (FLICA) Poly Caspase Assay Kit (Immunochemistry Technologies) all dilutions and staining protocols were performed according to the manufacturer’s instruction. Briefly, after 96 h of culture in Th0, Th1, Th2, Th17 or iTreg polarizing condition, sorted naïve CD4 + T cells were incubated with a 30 × FLICA solution for 1 h at 37 °C. Following incubation time, cells were washed with apoptosis wash buffer included in the kit. Cells were then analysed on a MoFlo flow cytometer (Beckman Coulter), gating on the live cells and measuring the fluorescence due to the presence of FAM-FLICA bound to several caspases (caspase-1, -3, -4, -5, -6, -7, -8 and -9). ELISA Mouse IL-4, IL-10, IL-17A, IFN-γ, GM-CSF, IL-23 and TGF-β 1 were measured using commercial kits (eBioscience). Mouse TGF-β 3 was measured using commercial kit (Catalog# SEB949Mu) from Cloud-clone. Briefly, ELISA plates were coated with 100 μl of anti-cytokine capture antibody at 4 °C overnight. Plates were then washed × 5 with 0.05% PBS-Tween (PBST) and coated for 1 h with the blocking buffer provided by the manufacturer. Samples or standards were added in duplicates (100 μl per well) and incubated at 4 °C overnight. Wells were washed × 5 with PBST and incubated with 100 μl of anti-cytokine detection antibody at 4 °C overnight. Wells were then washed × 5 with PBST and incubated with 100 μl of avidin-HRP at room temperature for 30 min. Thereafter, wells were washed × 7 with PBST and incubated with 100 μl per well of a substrate. The reaction was stopped after 15 min with 1 M H 2 SO 4 and absorbance was measured using a multiplate microplate fluorescence reader (Synergy HT, Biotek) at 405 nm. RNA extraction, real-time PCR and microarray analyses CD4 + T cells were isolated from WT mice (isolated with anti-biotin magnetic beads (Miltenyi Biotec), cultured in Th0, Th1, Th2 and iTreg polarizing conditions and used for microarray analyses and real-time PCR reactions. CD4 + T cells from 5C.C7 Rag2 −/− mice were cultured in Th0, Th1, Th2 and iTreg polarizing conditions and used exclusively for real-time PCR reactions. After 96 h of culture, cells were collected and RNA was extracted using the RNAqueous extraction kit according to the manufacturer’s protocols (Applied Biosystems). Briefly, cells were homogenized in lysis buffer (total volume of 0.5 ml) and passed through a column. After successive washes, RNA was eluted. For real-time PCR reactions, T-bet (Mm00450960_m1), GATA3 (Mm00484683_m1), STAT5a (Mm03053818_s1), STAT6 (Mm00447411_m1), ROR γ t (Mm01261022_m1), Foxp3 (Mm00475162_m1) and tryptophan hydroxylase-1 ( Tph1 ) (Mm00493794_m1) measurements were performed with Taqman primers and probes from Applied Biosystems. The housekeeping gene GAPDH (Mm99999915_g1) was used as control. Microarray analyses were performed using affymetrix genechip. Briefly, the cDNA (10 μg) was fragmented and labelled and then hybridized to a GeneChip Mouse Genome 430 2.1 array (Affymetrix). Affymetrix microarray data analysis was performed using Partek Genomics Suite software (Partek Inc.). Default settings were used for quantile normalization and RMA summarization. The samples were grouped and statistics were applied using the analysis of variance model employing linear contrast. Linear contrast was established for each pair of grouped samples for which the analysis was appropriate. Gene lists were then created for each analysis for downstream pathway analysis using threshold values of FDR-adjusted P -value ≤0.05 and fold change ≥2 and ≤2. The Ingenuity Pathways Analysis (Ingenuity Systems) applications were used to generate canonical pathways associated with the differentially expressed gene profiles extracted from the transcriptome data. RNA extraction from spinal cord tissue was performed using RNAqueous extraction kit according to the manufacturer’s protocol (Applied Biosystems). Briefly, 1 mg of spinal cord tissue was homogenized in lysis buffer (total volume of 0.5 ml) and passed through a column. After successive washes, RNA was eluted and reverse transcription was performed using i-Script cDNA synthesis kit (Bio-Rad Laboratories). PCR reactions were performed with IFN- γ (Mm01168134_m1) and IL-17A (Mm00439619_m1) Taqman primers and probes from Applied Biosystems. Relative gene expression was determined using the housekeeping gene GAPDH (Mm99999915_g1) as control. EAE mouse model EAE was induced in 8- to 10-week-old WT or IL-10 −/− mice using Hooke Labs EAE induction kit (EK-2110) according to the manufacturer’s instructions (Hooke Laboratories Inc.). Mice were scored daily on a scale of 0–5 in a double-blind manner with the following criteria: score 0, no signs of neurological disease; score 1, flaccid paralysis of the tail; partial or no tail muscle tone, mouse is unable to curl tail around finger or pencil; score 2, weak hindlimb paralysis or wobbling gait and/or impaired righting reflex; score 3, bilateral hindlimb paralysis, mouse drags its hindlimbs over flat surface and/or exhibits incontinence; score 4, hind- and forelimb paralysis, mouse barely moves around; score 5, moribund animal). For NAD + treatment, mice received a daily intraperitoneal injection (60 mg in 100 μl in PBS) or a placebo solution (100 μl of PBS) at the same day than MOG immunization. Mice were killed at day 18 and single-cell suspension was obtained from spleens for flow cytometry analysis. To test whether NAD + was able to reverse the development of EAE, another group of mice was treated daily (for a period of 10 days) with NAD + (60 mg per mouse) or a placebo solution (PBS) 15 days after MOG immunization when mice were scored 3 with a bilateral hindlimb paralysis. EAE disease progression was monitored. For Tph1 inhibition, mice were subjected to MOG immunization and treated daily with NAD + . One week after MOG immunization, mice received daily intraperitoneal injections (simultaneous to NAD + ) of p -Chlorophenylalanine (1 ml of a 10 mM stock solution, catalogue number 0938, Tocris Bioscience). Adoptive transfer Naïve sorted CD4 + CD25 − CD44 low CD62L high cells were cultured in Th1 polarizing in the presence of NAD + (250 μM), PBS or a cocktail of NAD + (250 μM) and Tph1 inhibitor (200 μM). After 4 days of culture, cells were collected, washed and 2 × 10 6 cells were re-suspended in 100 μl of PBS and injected intravenously in mice that were subjected to EAE at days 3, 6 and 9 post MOG-immunization. Histology, immunohistochemistry and quantification Animals used to assess EAE clinical symptoms ( n =6 per group) were killed 25 days after MOG immunization. After transcardial perfusion with 4% paraformaldehyde, lumbar spinal cord was isolated from the three groups of mice: (i) mice that were treated daily with a placebo solution (PBS), (ii) mice that were treated daily with NAD + and (iii) mice that were treated 15 days with NAD + after MOG immunization (when mice developed hindlimb paralysis). Spinal cords from the three groups were fixed in 4% paraformaldehyde for 24 h and processed for paraffin histology. Histological stainings with LFB (American MasterTech Scientific Inc.) and H&E (Sigma) were performed on 8-μm-thick transverse paraffin sections and immunohistochemistry was performed on 20-μm-thick paraffin sections. Primary antibodies used for immunohistochemistry were: monoclonal antibody to MBP (SMI-94) (1:400, Millipore) and rabbit polyclonal antibody to NF 200 (1:50, Sigma), Ki67 (1:30, Sigma) and Musashi (1:50, Millipore) followed by secondary detection with Alexa Fluor conjugates (Molecular Probes). DAPI (Vector Laboratories) was used to label nuclei. Brightfield and fluorescent images were obtained from an FSX100 microscope (Olympus). The areas of demyelination were quantified either by immunocytochemistry or immune fluorescence microcopy using ImagePro Plus 7.0 software (Media Cybernetics). For brightfield immunohistochemistry analysis, before quantification, each RGB image was converted into an image representing exclusively the saturation channel, and then the segmentation values established on a region of interest corresponding to the white matter in the untreated group was applied to all sections. The results represent optical density and area. Staining artefacts were removed manually following automatic quantification. Total areas measured represent three full transverse spinal cord sections per animal for each group. For fluorescence determination of NF+ area, monochrome images were analysed by quantifying intensity values using an automated segmentation script based on values obtained on the untreated group. Count of absolute number of lymphocytes C57BL/6 mice (8- to 10-week old) were administered daily 60 mg of NAD + or a placebo solution (PBS) intaperitoneally during 4 days. Blood and spleen were collected after 4 days of treatment. Absolute number of lymphocytes in the blood was determined using a haemocytometer (model 850 FS, Drew Scientific). To determine absolute lymphocyte number in spleens, cells were isolated and counted with a haemocytometer, then stained with anti-CD4 + , anti-CD3 + or anti-B220 + antibodies and percentages were determined by flow analysis. Statistical analysis Data are presented as the mean±s.d. Statistical analysis compared the groups with a two-tailed Student’s t- test or Mann–Whitney test were appropriate. Only P -values <0.05 were considered statistically significant. How to cite this article: Tullius, S. G. et al. NAD + protects against EAE by regulating CD4 + T cell differentiation. Nat. Commun. 5:5101 doi: 10.1038/ncomms6101 (2014).